Control of electronic conduction at an oxide heterointerface using surface polar adsorbates The interface between LaAlO 3 and SrTiO 3 possesses a range of intriguing properties, notably a proposed connection between the surface state of the LaAlO 3 and the conductivity buried in the SrTiO 3 . Here we study the effect of the surface adsorption of a variety of common laboratory solvents on the conductivity at the interface between LaAlO 3 and SrTiO 3 . We show that the application of chemicals such as acetone, ethanol, and water can induce a large change in the conductivity, and, in particular, an insulator to metal transition around the critical LaAlO 3 thickness. This phenomenon is observed only for polar solvents. These data provide experimental evidence for a general polarization-facilitated electronic transfer mechanism. The transfer of electrons between a solid surface and adsorbed atomic or molecular species is fundamental in natural and synthetic processes, being at the heart of most catalytic reactions and many sensors. In special cases, metallic conduction can be induced at the surface of, for example, Si-terminated SiC [1] , or mixed-terminated ZnO [2] , in the presence of a hydrogen adlayer. Generally, only the surface atoms are significantly affected by adsorbates. However, remotely changing electronic states far from the adsorbed layer is possible, if these states are electrostatically coupled to the surface. Here we show that the surface adsorption of common solvents such as acetone, ethanol, and water can induce a large change in the conductivity at the buried interface between SrTiO 3 substrates and LaAlO 3 thin films [3] , [4] , [5] , [6] , [7] , [8] , and an adsorbate induced insulator to metal transition was observed when the thickness of LaAlO 3 , d LAO , is around 3 unit cells (uc). This phenomenon is observed only for polar solvents. Our result provides experimental evidence that adsorbates at the LaAlO 3 surface induce accumulation of electrons at the LaAlO 3 /SrTiO 3 interface, suggesting a general polarization-facilitated electronic transfer mechanism, which can be adapted for use in a range of oxide-based devices. The intense interest in the LaAlO 3 /SrTiO 3 interface [3] , [4] , [5] , [6] , [7] , [8] , [9] , [10] , [11] , [12] , [13] , [14] , [15] , [16] , [17] , [18] , [19] , [20] , [21] , [22] has led to several recent experimental observations that suggest a close relationship between the interface and the LaAlO 3 surface. These include the use of conducting atomic force microscopy probes to toggle a metal insulator transition [10] , [11] , [12] through the writing of surface charge [12] , [13] , and the use of capping layers of SrTiO 3 (ref. 14 ) or SrCuO 2 (ref. 15 ) to alter the interface conductivity. The origin of these effects, and indeed the interface conductivity itself, remains in debate [4] , [16] , [17] , [18] , [19] , [20] , [21] , [22] . The transfer of electrons from the surface to the interface, to reconcile the polar discontinuity between the neutral {100} layers in SrTiO 3 and the charged layers in {100} LaAlO 3 , is one model that naturally connects the electronic states of the interface and LaAlO 3 surface [4] , [18] , [19] , [20] , [21] , [22] . However, despite these concepts and recent experimental progress, the effect of surface adsorbates has not been investigated. This issue is addressed in the present work. We have found that the exposure of LaAlO 3 /SrTiO 3 samples to a polar solvent can increase the sheet carrier density, n 2 d , by more than 2×10 13 cm −2 , representing a change of the same order as the total charge density typical in this system [5] , [6] , [7] , [8] . Compared with the strong perturbations associated with other surface processes, that is, the extremely strong local electric field produced by the conducting atomic force microscopy probes [10] , [11] , [12] , [13] , or the structural variation by introducing capping layers grown at high temperatures [14] , [15] , the changes associated with room-temperature treatment using these solvents would naively be expected to be small. However, such processes result in a surprisingly large modulation of n 2 d , revealing a dramatic surface-interface coupling. Transport characterization The fabrication of the conducting LaAlO 3 /SrTiO 3 interfaces and the surface adsorption process (SAP) are described in the Methods. 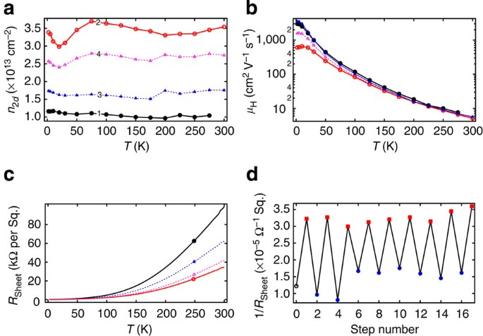Figure 1: Transport characterization. Temperature dependence of (a) Sheet carrier density,n2d, (b) Hall mobility,μH, and (c) Sheet resistance,RSheet, in different states of adLAO=10 uc LaAlO3/SrTiO3sample. The black closed circles represent the as-grown sample before experiencing any SAP. The red open circles represent the sample after an acetone SAP. The blue closed triangles represent the sample after heating atT=663 K in an O2pressure of 1.33×10−2Pa for 5 h. The pink open triangles represent the sample after a water SAP. The processing and measurement sequence follows the labelled order in (a). (d) Room-temperature conductivity, 1/Rsheet, of adLAO=10 uc LaAlO3/SrTiO3sample that was repeatedly processed by water SAP (red closed squares) and recovered by heating at 573 K in an oxygen flow for 3 h (blue closed circles). The black open circle represents the as-grown sample. As shown in Figure 1a , labels 1 & 2, a SAP using acetone increased n 2 d from ∼ 1×10 13 cm −2 to more than 3×10 13 cm −2 for a d LAO =10 uc sample, over a wide temperature range (2 K≤ T ≤300 K). This remarkable modulation suggests that the acetone molecules have been adsorbed on the LaAlO 3 surface and, in turn, change the electronic states at the buried interface. Heating the sample at T =380 K in a moderate vacuum (<10 3 Pa, with a helium background) for several hours produced negligible conduction change (not shown). However, the original sample state was recovered after heating at an elevated temperature of 653 K, evidenced by the decrease in n 2 d ( Fig. 1a , label 3) and the subsequent increase after another SAP using water ( Fig. 1a , label 4). These facts indicate that the surface adsorption is reversible but strong, not a physical adsorption driven by the relatively weak van der Waals force, and thus likely involves electron transfer. We note that as a function of n 2 d , the qualitative shape of the n 2 d ( T ) data at low temperatures is quite different. This is likely associated with the complex temperature and electric-field dependencies of SrTiO 3 , leading to a non-trivial variation of the confining potential as a function of n 2 d , as discussed elsewhere [23] . Figure 1: Transport characterization. Temperature dependence of ( a ) Sheet carrier density, n 2 d , ( b ) Hall mobility, μ H , and ( c ) Sheet resistance, R Sheet , in different states of a d LAO =10 uc LaAlO 3 /SrTiO 3 sample. The black closed circles represent the as-grown sample before experiencing any SAP. The red open circles represent the sample after an acetone SAP. The blue closed triangles represent the sample after heating at T =663 K in an O 2 pressure of 1.33×10 −2 Pa for 5 h. The pink open triangles represent the sample after a water SAP. The processing and measurement sequence follows the labelled order in ( a ). ( d ) Room-temperature conductivity, 1 /R sheet , of a d LAO =10 uc LaAlO 3 /SrTiO 3 sample that was repeatedly processed by water SAP (red closed squares) and recovered by heating at 573 K in an oxygen flow for 3 h (blue closed circles). The black open circle represents the as-grown sample. Full size image Accompanying the n 2 d increase, a striking reduction in the Hall mobility, μ H , from 3,000 cm 2 V −1 s −1 to 600 cm 2 V −1 s −1 ( T =2 K) is observed after the acetone SAP ( Fig. 1b ). μ H decreases quickly with increasing temperature, with a relatively small room temperature value of μ H ∼ 6 cm 2 V −1 s −1 due to the dominance of phonon scattering. At this temperature, μ H also has a very weak dependence on n 2 d , thus the conductivity 1 /R sheet is a reasonable and convenient index of n 2 d ( Fig. 1a, c ), and we will use it hereafter to characterize the effect of the SAP process on n 2 d for a variety of common solvents. To study the repeatability of the adsorption/desorption processes, we repeatedly performed water SAP on a LaAlO 3 /SrTiO 3 sample followed by a heating step at 573 K in an oxygen flow, to reset the system ( Fig. 1d ). The sample switches reproducibly between a high-conductivity state after SAP and a low-conductivity state after heating. Effect of SAP using different solvents To explore the origin of the SAP-induced n 2 d , we have studied the effect of SAP using a variety of solvents with d LAO =10 uc samples. These solvents can be classified into three categories: non-polar, polar aprotic (no dissociable H + ), and polar protic (dissociable H + ). 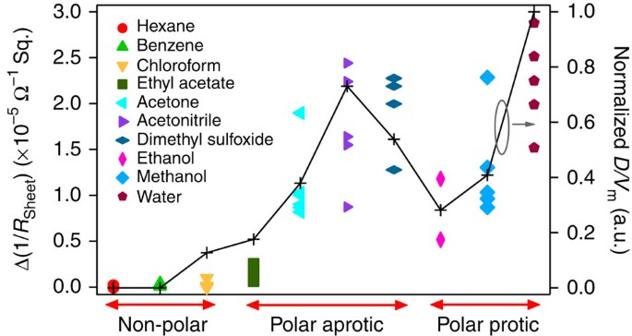Figure 2: Effect of SAP using different solvents. The difference in 1/Rsheetafter and before SAP, Δ(1/Rsheet), reflects the change inn2dat room temperature. A clear increase in Δ(1/Rsheet) is observed after SAP using polar solvents, independent of their aprotic or protic character. Δ(1/Rsheet) is reasonably scaled with the molecular dipole moment (D) of each solvent divided by the corresponding molecular volume (Vm) (crosses). The line is a guide to the eye. In each category, the solvents are ordered from left to right by increasing polarizability. At least two samples were used for each solvent and all samples weredLAO=10 uc and in the as-grown state before SAP. The results are summarized in Figure 2 . Clearly, SAP using non-polar solvents produces no significant modulation in 1/R sheet and by extension, n 2 d . SAP using a relatively weak polar solvent such as ethyl acetate produces a slight increase in n 2 d , whereas using more polar solvents produces a much larger increase, independent of whether the solvents are aprotic or protic. In Figure 2, we also show that Δ(1 /R Sheet ) is well scaled with the molecular dipole moment divided by the molecular volume. These results suggest that the polar nature of solvents has a key role in determining the magnitude of the observed changes for the different solvents. In the context of an electrostatic mechanism, the scaling of the change with the dipole moment density would be reasonable, as the strength of the effect should be related to not only the molecular dipole moment, but also the areal density of the molecules on the surface. Figure 2: Effect of SAP using different solvents. The difference in 1 /R sheet after and before SAP, Δ(1 /R sheet ), reflects the change in n 2 d at room temperature. A clear increase in Δ(1 /R sheet ) is observed after SAP using polar solvents, independent of their aprotic or protic character. Δ(1 /R sheet ) is reasonably scaled with the molecular dipole moment ( D ) of each solvent divided by the corresponding molecular volume ( V m ) (crosses). The line is a guide to the eye. In each category, the solvents are ordered from left to right by increasing polarizability. At least two samples were used for each solvent and all samples were d LAO =10 uc and in the as-grown state before SAP. Full size image Comparison between SAP and adsorption of solvent vapour Further insights into the origin of the SAP-induced n 2 d can be made by comparing the effect of SAP with the effect of adsorption from a solvent vapour. It is well known that a thin layer of water coats all hydrophilic surfaces under ambient conditions [24] . Until now the adsorption of water on LaAlO 3 , particularly on the AlO 2 -terminated LaAlO 3 surface, has been scarcely studied. A water-dipping study showed that, whereas La 2 O 3 is highly hygroscopic, LaAlO 3 only reacts weakly with water [25] . In contrast, the adsorption of water on Al 2 O 3 is well understood. It is known that Al 2 O 3 adsorbs 1 monolayer of water when the relative humidity (RH) is ∼ 35%, and more than 5 monolayers for RH >70% (refs 26 , 27 ). Thus, although these studies cannot be trivially extrapolated to the current heterostructures, we expect a thin layer of water with full coverage will coat the AlO 2 -terminated LaAlO 3 surface when the LaAlO 3 /SrTiO 3 sample is exposed to RH >70% air at room temperature. Such a surface layer has also been inferred from charge writing experiments [28] . Nonetheless, despite the existing water layer, we can still modulate the conductivity using the macroscopically large volumes of solvent in the SAP process. 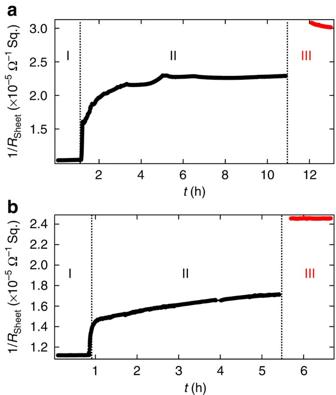Figure 3: Comparison between the effect of SAP and the effect of adsorption of solvent vapour. (a) Conductivity versus time plots for a sample exposed to (I) air of RH=30%, (II) air near the saturation point of water, and (III) followed by a water SAP. (b) Conductivity versus time plots for a sample exposed to (I) air of RH=30%, (II) air near the saturation point of acetone, and (III) followed by an acetone SAP. Note that surface adsorption of, for example, water, would have already taken place when the sample was kept in normal air. The exposure to the nearly saturated water (acetone) vapour for many hours should achieve a full and thicker coverage of adsorbates on the LaAlO3surface. The samples aredLAO=10 uc, and the measurements were performed at ambient environment. The irregular perturbations in (a) were caused by fluctuations in the local illumination and room temperature. Figure 3a shows that the conductivity of LaAlO 3 /SrTiO 3 is still sensitive to water SAP using liquid even after exposing it to water-saturated atmosphere for several hours. A similar result was found when acetone was used ( Fig. 3b ). From these results, we can conclude that the thickness of adsorbate layer also has an important role in the SAP effect, as the SAP with liquid is expected to produce a thicker adsorbed solvent film compared with the vapour experiments. Figure 3: Comparison between the effect of SAP and the effect of adsorption of solvent vapour. ( a ) Conductivity versus time plots for a sample exposed to (I) air of RH=30%, (II) air near the saturation point of water, and (III) followed by a water SAP. ( b ) Conductivity versus time plots for a sample exposed to (I) air of RH=30%, (II) air near the saturation point of acetone, and (III) followed by an acetone SAP. Note that surface adsorption of, for example, water, would have already taken place when the sample was kept in normal air. The exposure to the nearly saturated water (acetone) vapour for many hours should achieve a full and thicker coverage of adsorbates on the LaAlO 3 surface. The samples are d LAO =10 uc, and the measurements were performed at ambient environment. The irregular perturbations in ( a ) were caused by fluctuations in the local illumination and room temperature. Full size image LaAlO 3 thickness dependence A key feature of the LaAlO 3 /SrTiO 3 interface is that there exists a critical LaAlO 3 thickness, d LAO ∼ 4 uc, below which the interface is insulating [5] . It is instructive to see the dependence of the effect of SAP on the LaAlO 3 thickness. 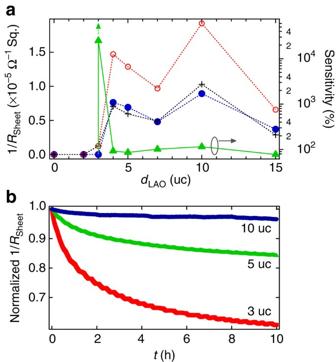Figure 4: LaAlO3thickness dependence. (a) The effect of SAP on samples of different LaAlO3thicknesses. The blue closed circles represent 1/Rsheetof the as-grown samples. The red open circles represent 1/Rsheetof the samples after an acetone SAP. The difference after and before acetone SAP, Δ(1/Rsheet), is represented by black crosses. Sensitivity (green triangles) was defined as a ratio between Δ(1/Rsheet) and 1/Rsheet(as grown). The green arrow indicates the measurement limit. ThedLAO=0 uc sample is a bare SrTiO3substrate. The acetone SAP triggers a transition from an insulating state to a conducting state for adLAO=3 uc sample. (b) The time dependence of 1/Rsheetafter acetone SAP fordLAO=3, 5, and 10 uc samples. All measurements were performed at ambient environment. The small perturbations in the data, notably on the 3 uc curve, were caused by small fluctuations in the room temperature. Lines are guides for the eye. As shown in Figure 4a , for d LAO =2 uc sample and bare SrTiO 3 substrate, no modulation in the conductivity is observed. For d LAO =3 uc, the as-grown sample is insulating and the acetone SAP drives the sample from an insulating state to a conducting state. In this case, the absolute modulation in the carrier density, as indexed by Δ(1 /R Sheet ), is smaller than that in the thicker samples, but the sensitivity, defined as the ratio of the conductivity change with respect to that of the as-grown sample, is much larger. We speculate that, with suitable optimization, this large sensitivity may be exploited for sensor applications. Figure 4: LaAlO 3 thickness dependence. ( a ) The effect of SAP on samples of different LaAlO 3 thicknesses. The blue closed circles represent 1 /R sheet of the as-grown samples. The red open circles represent 1 /R sheet of the samples after an acetone SAP. The difference after and before acetone SAP, Δ(1 /R sheet ), is represented by black crosses. Sensitivity (green triangles) was defined as a ratio between Δ(1 /R sheet ) and 1 /R sheet (as grown). The green arrow indicates the measurement limit. The d LAO =0 uc sample is a bare SrTiO 3 substrate. The acetone SAP triggers a transition from an insulating state to a conducting state for a d LAO =3 uc sample. ( b ) The time dependence of 1 /R sheet after acetone SAP for d LAO =3, 5, and 10 uc samples. All measurements were performed at ambient environment. The small perturbations in the data, notably on the 3 uc curve, were caused by small fluctuations in the room temperature. Lines are guides for the eye. Full size image Figure 4b shows the time-dependent 1/R sheet , immediately after an acetone SAP, of LaAlO 3 /SrTiO 3 samples of different LaAlO 3 thicknesses. As d LAO decreases, 1/R sheet tends to relax more quickly, indicating solvent desorption. This observation suggests that the surface adsorption is directly related to the nature of the LaAlO 3 surface, or its polar character. We note that a somewhat analogous observation has previously been found for the charge stability on the LaAlO 3 surface in the same system [12] . Next, we discuss the possible mechanisms that may explain these data. We exclude electrostatic attraction because the polar adsorbates themselves are charge-neutral as a whole and will not change the electrostatic boundary condition of LaAlO 3 /SrTiO 3 without the transfer of electrons [29] . Oxygen vacancies in the SrTiO 3 (ref. 16 ), atomic interdiffusion [17] , and an electronic reconstruction [4] , [18] , [19] , [20] have all been suggested to be the origin of the interfacial conductivity in the LaAlO 3 /SrTiO 3 system. In the case of the SAP experiments, we exclude the first two of these as we assume that a SAP at room temperature does not cause significant atomic structure changes at the interface, and we focus on the electronic reconstruction mechanism. 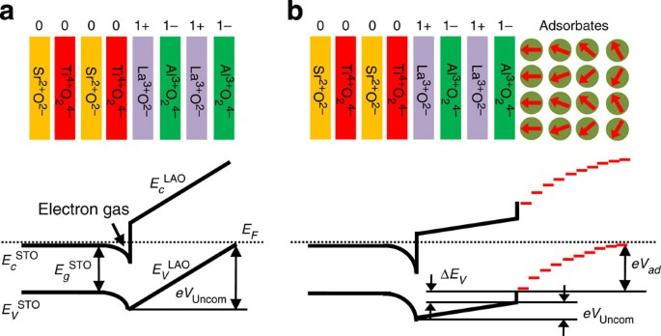Figure 5: Sketches of band diagrams and electron transfer mechanisms. (a) Idealized surface. Electrons transfer fromEVLAOof the LaAlO3surface to the conduction band of SrTiO3,ECSTO, near the interface.eVUncomroughly equals toEgSTO. (b) Surface with aligned polar adsorbates. Electrons transfer from the surface adsorbates toECSTOnear the interface. The built-in potential across the adsorbates,Vad, effectively reducesVUncomacross the LaAlO3layer. In both (a,b) bulk stoichiometry and valences are shown for simplicity. As discussed in several papers [19] , [20] , and illustrated in Figure 5a , for an idealized LaAlO 3 surface free from surface states, the valence band of LaAlO 3 , E V LAO is the electron source for the interface electrons. Here we assume no conductivity in the LaAlO 3 film itself, and, for simplicity, do not consider other processes that do not affect the electrostatic state of the LaAlO 3 . An uncompensated potential, V Uncom , across the LaAlO 3 film of the order of the band gap of SrTiO 3 , E g STO is needed to align the chemical potential over the whole structure. A simple electrostatic consideration shows that , where σ 0 is the charge density of one atomic layer, σ Inter is the total sheet electron density at the interface, e is the unit charge, and ɛ LAO is the dielectric constant of LaAlO 3 . In reality, σ Inter is larger than n 2 d because of the trapping of some electrons at the interface [19] . Immediately, we find that This simple relationship predicts the same thickness dependence of σ Inter as several more detailed theoretical calculations [20] , [30] , noting that V Uncom is fixed for an ideal surface. In the work presented here, d LAO is fixed, and the SAP induced change in n 2 d is thus associated with a reduction in V Uncom . Figure 5: Sketches of band diagrams and electron transfer mechanisms. ( a ) Idealized surface. Electrons transfer from E V LAO of the LaAlO 3 surface to the conduction band of SrTiO 3 , E C STO , near the interface. eV Uncom roughly equals to E g STO . ( b ) Surface with aligned polar adsorbates. Electrons transfer from the surface adsorbates to E C STO near the interface. The built-in potential across the adsorbates, V ad , effectively reduces V Uncom across the LaAlO 3 layer. In both ( a , b ) bulk stoichiometry and valences are shown for simplicity. Full size image We note that there are several possibilities of reduction of V Uncom . In practice, all samples have surface states associated with inevitable defects, surface reconstructions, surface adsorbates and so on. If these surface states are within the bandgap of LaAlO 3 , they can replace E V LAO as more energetically favourable electron sources, where a relatively smaller V Uncom is required to dope electrons into the SrTO 3 . As far as surface adsorbates are concerned, they may interact with surface atoms or oxygen defects, and cause complex surface states. Two recent theoretical papers have suggested that the dissociation of hydrogen [21] and redox reactions [22] on the LaAlO 3 surface as possible electron sources. In both cases, V Uncom is reduced compared with that of the idealized surface. The role of water on the LaAlO 3 surface has also been recently stressed in theoretical calculations by S. Hellberg (personal communication). However, we caution that the observed accumulation of electrons by SAP cannot be fully explained by adsorbate-induced surface states alone, because the polar character of the adsorbates and their thickness were found to have a vital role in our experimental results. With the above picture in mind, we can interpret our results as follows: the strong polarization in the LaAlO 3 layer aligns to a degree the polar adsorbates nearest the surface, with a decaying trend as we move away into the adsorbate layer. As shown schematically in Figure 5b , this leads to an electrostatic potential across the adsorbate layer, V ad , quite similar to the built-in potential in the polar LaAlO 3 . As a result, electrons are sourced from the adsorbates instead of E V LAO of the surface LaAlO 3 to the LaAlO 3 /SrTiO 3 interface, and V Uncom across the LaAlO 3 is effectively decreased. σ Inter increases according to Equation (1), consistently explaining the observed SAP-induced accumulation of electrons at the LaAlO 3 /SrTiO 3 interface. In this picture, the change in σ Inter is proportional to the value of V ad and the areal density of adsorbates. If we assume that the thickness of the adsorbate layer is the same for all solvents, and that all solvents are equally likely to transfer electrons it is simple to show that Δ σ Inter will be proportional to D/V m , consistent with the experimentally observed scaling relation between Δ(1 /R Sheet ) and D/V m ( Fig. 2 ). Our present observation is quite distinct from the proposed water-cycle mechanism that accounts for the modulation of interface conductivity by biased conductive scanning probe, because we achieve conductivity changes without actively dissociating water molecules [28] . We note that in principle the biased scanning probe will also change the physical distribution of the adsorbates, (for example, water), in addition to chemical changes, which may also contribute to the modulation in the interface conductivity in the charge writing experiments [10] , [11] , [12] , [13] . The observed close coupling between polar surface adsorbates and interface conductivity provides new insights into the origin of the electron gas at the LaAlO 3 /SrTiO 3 interface, and demonstrates a new tuning parameter in controlling this state, which has the potential to be applied broadly in a wide range of novel oxide-based devices. These data also suggest that many of the conflicting (and often contradictory) studies of this popular system can be explained by this observation, that is, whether measurements are made in situ [31] , or after various surface exposures (for example, atmospheric water, or solvent cleaning) [32] , [33] , [34] , the sensitive electronic structure of the interface may be dramatically altered. For example, the predicted electric field across the LaAlO 3 layer [18] , [19] , [20] was not observed in X-ray photoemission studies [32] that may be explained consistently because the surface adsorbates (in particular atmospheric water) induced by the ex-situ processing reduce V Uncom , or equally, the electrical field across the LaAlO 3 layer. In contrast, in the LaAlO 3 /SrTiO 3 superlattices of multiple interfaces, the interfaces relatively far away from the surface may not be significantly affected by adsorbates [34] . Sample fabrication Using optical lithography and lift-off, a six-contact Hall bar (central bar length 50 μm, width 10 μm) with amorphous AlO x as a hard mask was patterned onto the atomically flat TiO 2 -terminated SrTiO 3 (100) substrates. The LaAlO 3 thin films were grown on the patterned substrates by pulsed laser deposition with the growth monitored by in-situ reflection high-energy electron diffraction. The conducting interfaces are confined within the Hall bar region. For the samples shown in this article, the growth was at 923 K in an O 2 pressure of 1.33×10 −3 Pa, after a pre-annealing at 1,223 K in an O 2 pressure of 6.67×10 −4 Pa for half an hour. After deposition, there followed a post-annealing step at 873 K in an O 2 pressure of 4×10 4 Pa for one hour. During deposition, the laser repetition was 1 Hz and the laser energy density was 0.6 Jcm −2 . The same phenomenology is found for samples grown in a variety of temperatures, oxygen pressures and laser conditions. Electrical contact and measurement The conducting interface was contacted by ultrasonic bonding with Al wire. The temperature-dependent sheet resistance, sheet carrier density and mobility were deduced from standard transport measurements using the patterned Hall bar. All transport measurements were carried out using a standard four-probe method. To test for the possibility of parallel conductivity through the adsorbate layer itself, contacts were made directly to the surface using silver epoxy. No significant surface conduction was detected both before and after SAP, clearly demonstrating that the conduction is at all times dominated by the LaAlO 3 /SrTiO 3 interface. Surface adsorption process SAP was achieved by placing a drop of the liquid solvent on the sample surface at room temperature and blowing off all visible solvent within less than 10 s using dry nitrogen gas. Contacts were either left on the samples during the SAP, or reconnected afterwards; no significant difference in the conduction was observed by using either method. How to cite this article: Xie Y. et al . Control of electronic conduction at an oxide heterointerface using surface polar adsorbates. Nat. Commun. 2:494 doi: 10.1038/ncomms1501 (2011).